hESC-derived Olig2+progenitors generate a subtype of astroglia with protective effects against ischaemic brain injury Human pluripotent stem cells (hPSCs) have been differentiated to astroglia, but the utilization of hPSC-derived astroglia as cell therapy for neurological diseases has not been well studied. Astroglia are heterogeneous, and not all astroglia are equivalent in promoting neural repair. A prerequisite for cell therapy is to derive defined cell populations with superior therapeutic effects. Here we use an Olig2-GFP human embryonic stem cell (hESC) reporter to demonstrate that hESC-derived Olig2 + progenitors generate a subtype of previously uncharacterized astroglia (Olig2PC-Astros). These Olig2PC-Astros differ substantially from astroglia differentiated from Olig2-negative hESC-derived neural progenitor cells (NPC-Astros), particularly in their neuroprotective properties. When grafted into brains subjected to global ischaemia, Olig2PC-Astros exhibit superior neuroprotective effects and improved behavioural outcome compared to NPC-Astros. Thus, this new paradigm of human astroglial differentiation is useful for studying the heterogeneity of human astroglia, and the unique Olig2PC-Astros may constitute a new cell therapy for treating cerebral ischaemia and other neurological diseases. Astroglia are a major cellular constituent in the central nervous system (CNS) and have crucial roles in neuronal development and function and in brain integrity [1] . Human astroglia have been efficiently derived from human pluripotent stem cells (hPSCs), including human embryonic stem cells (hESCs) and induced pluripotent stem cells (iPSCs) [2] , [3] . However, the utility of hPSC-derived astroglia as cell therapy for neurological diseases has not been explored. Ischaemic stroke is a major cause of mortality and disability. No effective therapy is currently available to promote recovery following cerebral ischaemia [4] . There is a strong rationale for pursuing hPSC-derived astroglia as a therapeutic candidate for ischaemic brain injury. It has long been known that transplanted immature astrocytes suppress glia scar formation and are beneficial to the lesioned CNS [5] , [6] . Dysfunction of astrocytes occurs during ischaemic injury to the CNS and contributes importantly to delayed neuronal damage [7] . Accumulating evidence shows that astroglial transplants derived from foetal tissue can be neuroprotective to the disordered CNS [8] , [9] . A recent study [10] further shows that transplanted human iPSC-derived neural progenitors can improve neurological function after brain ischaemia, probably as a consequence of a neurotrophic effect from astrocytes, rather than differentiation of the transplanted cells to neurons. Astroglia cells exhibit marked phenotypic heterogeneity. Different subtypes of astrocytes have been recognized based on different morphology, growth rates [11] , gene expression profiles [12] , electrophysiological properties [13] , gap junction coupling and calcium wave propagation dynamics [14] . A key prerequisite for astroglia-based therapeutic application of hPSCs is the derivation of defined cell populations in high purity. Previous transplantation studies have also shown that not all astrocytes are equivalent in their ability to promote repair [6] , [9] , [15] . To achieve optimal outcome of cell therapy, it is important to investigate whether specific populations of astroglia can be derived from purified populations of human neural progenitors and whether these astroglia are of better use than heterogeneous glial populations. The basic helix-loop-helix transcription factor Olig2 is required for motoneuron and oligodendrocyte development in mice [16] . Recent studies in rodents also show that Olig2 is expressed in neural progenitors and has important roles in astrocyte development. A subpopulation of cortical NPCs including radial glial cells at embryonic stages and GFAP + progenitor cells in the postnatal subventricular zone (SVZ) [17] , [18] , [19] are shown to express Olig2. Studies using a dominant-negative form of Olig2 indicate that Olig2 in postnatal SVZ NPCs directs them to differentiate to cortical astrocytes [20] . Olig2 + progenitor cells in the spinal cord can also give rise to a subset of astrocytes [21] , [22] , and immunoreactive nuclear Olig2 is present in astrocytes in the grey matter of the normal adult mouse spinal cord [23] . During astrocyte development, Olig2 is transiently expressed in immature astrocytes at neonatal stages, and its level is progressively downregulated in astrocytes at late postnatal stages. Furthermore, by using a spatiotemporally specific conditional ablation approach, Olig2 is shown to have a crucial role in astrocyte development in the entire CNS, particularly in the white matter [24] . Although accumulative evidence from rodents shows the importance of Olig2 for astroglia development, it is unknown whether Olig2 + progenitor cells in humans can generate astroglia. In this study, using Olig2-GFP knockin hESCs, in which GFP is inserted into the Olig2 gene locus so that ESC-derived cells that express Olig2 also express GFP [25] , [26] , we generate human astroglia from Olig2 − /GFP − (negative) NPCs and Olig2 + /GFP + (positive) progenitor cells (Olig2PCs). We refer to them as NPC-astroglial cells (NPC-Astros) and Olig2PC-astroglial cells (Olig2PC-Astros), respectively. We demonstrate that Olig2PC-Astros exhibit a number of key differences in functions and gene expression profiles from NPC-Astros in vitro . Furthermore, upon transplantation into the brain of rats after global cerebral ischaemia (GCI), both Olig2PC-Astros and NPC-Astros significantly protect neurons in the CA1 region, but rats that received Olig2PC-Astros show better performance in the water-maze test compared to rats that received NPC-Astros. Thus, two defined subtypes of astroglia generated from hESC-derived Olig2-positive versus Olig2-negative neural progenitors, exhibit distinct properties and neuroprotective effects. Olig2PCs generate astroglial cells in the presence of BMP4 We employed an Olig2-GFP hESC reporter to study human astroglial differentiation. Based on our previous studies [26] , after being treated with retinoic acid (RA) and the sonic hedgehog agonist purmorphamine (Pur), Olig2-GFP hESCs were efficiently differentiated to Olig2PCs ( Fig. 1a ). The GFP + colonies at day 20 were disaggregated to single cells and subjected to FACS. As shown in Fig. 1b , FACS analysis indicated that the percentage of Olig2 + /GFP + cells increased from 0.19±0.1% at day 0 to 55.8±4.9% at day 20 ( n =5). To assess the composition of Olig2PCs, we stained the cells 2 days after FACS with a panel of markers. As shown in Fig. 1d , nearly all of the cells were positive for GFP (98.5±0.6%, n =3), Olig2 (98.1±0.9%, n =3), glial precursor marker A2B5 (97.5±2.4%, n =3) and the neural stem cell marker nestin (97.3±1.5%, n =3). Few βIII-tubulin-positive neurons (<1%) were identified 2 days after FACS, but they were not observed after two to three passages in the culture ( Supplementary Fig. S1 ). None of the cells was positive for the oligodendrocyte progenitor cell (OPC) markers NG2 and PDGFRα, nor for the astrocyte marker GFAP at this stage ( Supplementary Fig. S1 ). To examine whether the Olig2PCs could generate astroglia, we cultured FACS-purified Olig2PCs in the presence of bone morphogenetic protein 4 (BMP4), which promotes astrocyte lineage commitment in vivo [27] . We observed that, after 4-day culture in the presence of BMP4, GFAP expression was undetectable, but another astrocyte marker S100β was strongly expressed ( Supplementary Fig. S2a ). These S100β + cells could also be labelled by anti-GFP staining ( Supplementary Fig. S2b ), indicating that they were derived from GFP + Olig2PCs. As shown in Fig. 1f , after 20-day culture in the presence of BMP4, nearly all the cells had become positive for GFAP (94.4±3.4%, n =3) and S100β (95.9±1.5%, n =3). The putative glial precursor marker A2B5 was also expressed in many of the cells (77.0±7.6%, n =3). When exposed to a culture medium containing 10% foetal bovine serum (FBS), these cells became negative for A2B5 but were still positive for GFAP (97.6±1.8%, n =3) and S100β (97.1±1.9%, n =3) ( Fig. 1f ). Under the xeno-free culture conditions, nearly all the cells expressed both CD44, a marker used to identify astrocyte-restricted precursor cells [28] , and vimentin, a major cytoskeletal protein expressed in immature astrocytes [29] ( Fig. 1h , 96.3±2.4% and 99.6±0.1% of the total cells were positive for CD44 and vimentin, respectively, n =3 for both). The robust expression of CD44 and vimentin indicated that the hESC-derived astroglia were immature, rather than mature astrocytes. As shown in Fig. 1j , RT-PCR results also confirmed the expression of CD44, GFAP and the astrocyte-specific glutamate transporter GLAST in the cells. The Olig2 transcript was not detectable from all the cells, and GFP signal was absent. Ciliary neurotrophic factor (CNTF) was also used to induce astroglia differentiation from hPSCs [2] , [3] . We found that after being cultured in the presence of CNTF for 20 days, these Olig2PCs were induced to GFAP + astroglia and similarly, Olig2 expression was also terminated ( Supplementary Fig. S3 ). 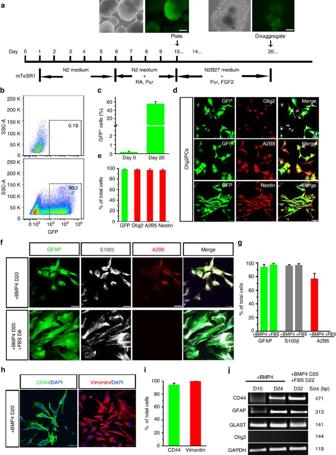Figure 1: Highly efficient differentiation of astroglial cells from Olig2PCs. (a) A schematic procedure for differentiating Olig2-GFP hESCs to Olig2+/GFP+progenitor cells or ‘Olig2PCs’. Insets: left, bright field and GFP channel demonstrating that many EBs show GFP fluorescence at day 10 with the treatment of RA and Pur. Right, bright field and GFP channel showing that at day 20, the EBs become flat after plating and many cells show GFP fluorescence. These colonies are ready to be disaggregated and subjected to FACS. Scale bars represent 300 μm. (bandc) FACS analysis showing the percentage of GFP+cells at day 0 and day 20 during differentiation (n=5). (dande) Representatives and quantification of GFP−, Olig2−, A2B5− and nestin-expressing cells 2 days after FACS (n=3). (fandg) Representatives and quantification of GFAP−, S100β−, and A2B5-expressing cells when the Olig2PCs are induced to astroglia by BMP4 or FBS (n=3). (handi) Representatives and quantification of CD44- and vimentin-expressing cells when cultured with medium containing BMP4 (n=3). (j) RT-PCR data showing expression of CD44 (471 bp), GFAP (313 bp), GLAST (141 bp) and Olig2 (144 bp) in Olig2PC-Astros cultured with BMP4 or FBS. Data are presented as means±s.e.m. Blue, DAPI-stained nuclei. Scale bars in all panels represent 50 μm. Figure 1: Highly efficient differentiation of astroglial cells from Olig2PCs. ( a ) A schematic procedure for differentiating Olig2-GFP hESCs to Olig2 + /GFP + progenitor cells or ‘Olig2PCs’. Insets: left, bright field and GFP channel demonstrating that many EBs show GFP fluorescence at day 10 with the treatment of RA and Pur. Right, bright field and GFP channel showing that at day 20, the EBs become flat after plating and many cells show GFP fluorescence. These colonies are ready to be disaggregated and subjected to FACS. Scale bars represent 300 μm. ( b and c ) FACS analysis showing the percentage of GFP + cells at day 0 and day 20 during differentiation ( n =5). ( d and e ) Representatives and quantification of GFP−, Olig2−, A2B5− and nestin-expressing cells 2 days after FACS ( n =3). ( f and g ) Representatives and quantification of GFAP−, S100β−, and A2B5-expressing cells when the Olig2PCs are induced to astroglia by BMP4 or FBS ( n =3). ( h and i ) Representatives and quantification of CD44- and vimentin-expressing cells when cultured with medium containing BMP4 ( n =3). ( j ) RT-PCR data showing expression of CD44 (471 bp), GFAP (313 bp), GLAST (141 bp) and Olig2 (144 bp) in Olig2PC-Astros cultured with BMP4 or FBS. Data are presented as means±s.e.m. Blue, DAPI-stained nuclei. Scale bars in all panels represent 50 μm. Full size image Previously reported astroglia are derived from Olig2 − NPCs In previously reported protocols of astroglial differentiation, hPSCs were first differentiated to NPCs and then to astroglia [2] , [3] , [30] , [31] . Whether Olig2 is expressed at any stage of this astroglial differentiation procedure is unclear. We thus employed the Olig2-GFP transgene reporter to mark Olig2 expression using the reported protocol for astroglial differentiation by monitoring GFP fluorescence. 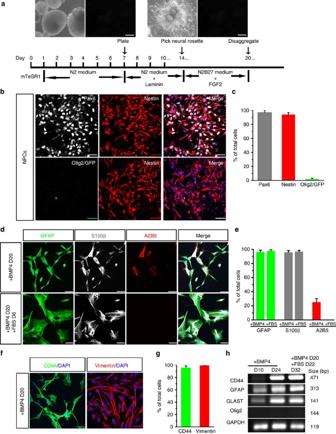Figure 2: Differentiation of astroglial cells from Olig2-negative NPCs. (a) A schematic procedure for differentiating Olig2-GFP hESCs to NPCs. Insets: left, bright field and GFP channel demonstrating that GFP fluorescence is undetectable at day 7 in the absence of RA and Pur. Right, bright field and GFP channel showing that at day 14, the EBs become flat after plating and neural rosettes were observed, but GFP fluorescence is undetectable. These neural rosettes are ready to be manually picked up and further cultured in suspension. Scale bars represent 300 μm. (bandc) Representative and quantification of Pax6, nestin, and Olig2/GFP-expressing cells among the cells disaggregated from neurospheres at D20 (n=3). Noticeably, very few cells are Olig2+/GFP+. (dande) Representative and quantification of GFAP-, S100β-, and A2B5-expressing cells when the NPCs are induced to astroglia by BMP4 or FBS (n=3). (fandg) Representatives and quantification of CD44- and vimentin-expressing cells when cultured with medium containing BMP4 (n=3). (h) RT-PCR data showing expressions of CD44 (471 bp), GFAP (313 bp), GLAST (141 bp) and Olig2 (144 bp) in NPC-Astros cultured with BMP4 or FBS. Data are presented as mean±s.e.m. Blue, DAPI-stained nuclei. Scale bars in all panels represent 50 μm. Figure 2a shows the differentiation protocol. From days 0 to 7, the Olig2-GFP hESCs formed embryoid bodies (EBs). Without exposure to RA and Pur, these EBs did not show GFP fluorescence, indicating the absence of Olig2 expression ( Fig. 2a inset). At day 20, the neurospheres were disaggregated and plated as single cells. As shown in Fig. 2b , nearly all the cells expressed the NPC markers, Pax6 (96.7±3.2%, n =3) and nestin (94.1±2.6%, n =3). However, very few of them (2.0±1.3%, n =3) were positive for Olig2/GFP in the absence of RA and Pur. To further differentiate the NPCs to astroglia, the NPCs were cultured in the presence of BMP4 for another 20 days. As shown in Fig. 2d , at this stage, nearly all of the cells expressed GFAP (96.4±2.3%, n =3) and S100β (95.8±2.4%, n =3), but continued to be GFP-negative. A2B5 was expressed in a subset of GFAP + /S100β + cells (25.4±4.8%, n =3). When these GFAP + cells were exposed to FBS, they became negative for A2B5 but continued to express GFAP (97.9±1.5%, n =3) and S100β (96.9 ±1.7%, n =3) ( Fig. 2e ). Nearly all of the cells were positive for CD44 and vimentin under the xeno-free culture condition ( Fig. 2f , 95.8±3.1% and 99.4±0.2% of total cells were positive for CD44 and vimentin, respectively, n =3 for both). As shown in Fig. 2h , RT-PCR results also confirmed the expression of CD44, GFAP and GLAST, the and absence of Olig2 in the cells. Figure 2: Differentiation of astroglial cells from Olig2-negative NPCs. ( a ) A schematic procedure for differentiating Olig2-GFP hESCs to NPCs. Insets: left, bright field and GFP channel demonstrating that GFP fluorescence is undetectable at day 7 in the absence of RA and Pur. Right, bright field and GFP channel showing that at day 14, the EBs become flat after plating and neural rosettes were observed, but GFP fluorescence is undetectable. These neural rosettes are ready to be manually picked up and further cultured in suspension. Scale bars represent 300 μm. ( b and c ) Representative and quantification of Pax6, nestin, and Olig2/GFP-expressing cells among the cells disaggregated from neurospheres at D20 ( n =3). Noticeably, very few cells are Olig2 + /GFP + . ( d and e ) Representative and quantification of GFAP-, S100β-, and A2B5-expressing cells when the NPCs are induced to astroglia by BMP4 or FBS ( n =3). ( f and g ) Representatives and quantification of CD44- and vimentin-expressing cells when cultured with medium containing BMP4 ( n =3). ( h ) RT-PCR data showing expressions of CD44 (471 bp), GFAP (313 bp), GLAST (141 bp) and Olig2 (144 bp) in NPC-Astros cultured with BMP4 or FBS. Data are presented as mean±s.e.m. Blue, DAPI-stained nuclei. Scale bars in all panels represent 50 μm. Full size image Comparison between Olig2PC-Astros and NPC-Astros Although similar in cell marker expression, Olig2PC-Astros differed substantially from NPC-Astros in morphology when cultured in adhesion in the presence of BMP4. As shown in Fig. 3a , Olig2PC-Astros exhibited a flat morphology, whereas NPC-Astros had a more compact and elongated morphology. When grown to high density, both types of cells tended to aggregate and form spheres ( Fig. 3a ). When hESC-derived neurons were plated onto the astroglia, both Olig2PC-Astros and NPC-Astros were supportive for neuronal survival and neurite formation ( Fig. 3a ). 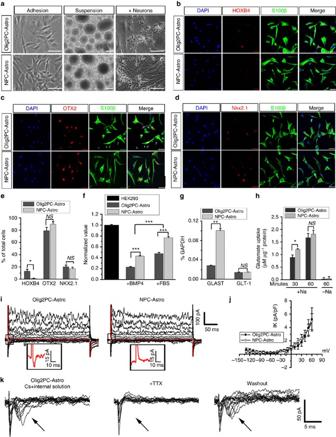Figure 3: Characterization of Olig2PC-Astros and NPC-Astros. (a) Left panels, representative Olig2PC-Astros and NPC-Astros cultured in adhesion. Notice the different morphology of the two types of astroglial cells. Middle panels, representative Olig2PC-Astros and NPC-Astros cultured in suspension. Right panels, representatives showing that both Olig2PC-Astros and NPC-Astros are supportive for the growth of hESC-derived neurons. Scale bars represent 250 μm. (b–d) The expression of HOXB4, OTX2 and NKX2.1 in S100β+Olig2-Astros and NPC-Astros. Blue, DAPI-stained nuclei. Scale bars represent 50 μm. (e) Quantification of HOXB4-, OTX2- and NKX2.1-expressing cells in Olig2-Astros and NPC-Astros (n=4). (f) Quantitative analysis of the proliferation rate of Olig2PC-Astro and NPC-Astros relative to HEK 293 cells. Notice that NPC-Astros proliferate more robustly than Olig2PC-Astros when cultured with either BMP4 or FBS (n=4). (g) Quantitative PCR analysis of GLAST and GLT-1 mRNA expression in Olig2PC-Astros and NPC-Astros (n=3). (h) Glutamate uptake analysis showing that both types of astroglia were capable of glutamate uptake. Notice that NPC-Astros showing glutamate uptake at a higher rate at the 30-min time point than Olig2PC-Astros (n=4). This uptake capability is Na+-dependent and can be abolished by the Na+-free solution. (i) Voltage steps (clamped at −70 mV and stepped from −130 to +60 mV at 10 mV increments for 300 ms) induced outward currents in both Olig2PC-Astros and NPC-Astros. A small inward current is detected in some Olig2PC-Astros (6 out of 10) but not in NPC-Astros shown by the traces highlighted in red and enlarged in the insets. The traces are presented after leak subtraction to reveal the voltage-gated currents. (j) Current-voltage relationship of the outward currents. (k) Using Cs+internal solution, the outward current is eliminated. The inward currents in Olig2PC-Astros are then recorded with the cells held at −70 mV. To maximally activate the inward currents, a 100-ms preconditioning pulse at −100 mV is delivered to the recorded cells before voltage steps (stepped from −70 to +50 mV at 10 mV increments for 50 ms). The representative traces show that the inward currents are reversibly blocked by TTX. The traces are presented after leak subtraction. Student’st-test, *P<0.05, **P<0.01 and ***P<0.001. NS represents no significance. Data are presented as mean±s.e.m. Figure 3: Characterization of Olig2PC-Astros and NPC-Astros. ( a ) Left panels, representative Olig2PC-Astros and NPC-Astros cultured in adhesion. Notice the different morphology of the two types of astroglial cells. Middle panels, representative Olig2PC-Astros and NPC-Astros cultured in suspension. Right panels, representatives showing that both Olig2PC-Astros and NPC-Astros are supportive for the growth of hESC-derived neurons. Scale bars represent 250 μm. ( b – d ) The expression of HOXB4, OTX2 and NKX2.1 in S100β + Olig2-Astros and NPC-Astros. Blue, DAPI-stained nuclei. Scale bars represent 50 μm. ( e ) Quantification of HOXB4-, OTX2- and NKX2.1-expressing cells in Olig2-Astros and NPC-Astros ( n =4). ( f ) Quantitative analysis of the proliferation rate of Olig2PC-Astro and NPC-Astros relative to HEK 293 cells. Notice that NPC-Astros proliferate more robustly than Olig2PC-Astros when cultured with either BMP4 or FBS ( n =4). ( g ) Quantitative PCR analysis of GLAST and GLT-1 mRNA expression in Olig2PC-Astros and NPC-Astros ( n =3). ( h ) Glutamate uptake analysis showing that both types of astroglia were capable of glutamate uptake. Notice that NPC-Astros showing glutamate uptake at a higher rate at the 30-min time point than Olig2PC-Astros ( n =4). This uptake capability is Na + -dependent and can be abolished by the Na + -free solution. ( i ) Voltage steps (clamped at −70 mV and stepped from −130 to +60 mV at 10 mV increments for 300 ms) induced outward currents in both Olig2PC-Astros and NPC-Astros. A small inward current is detected in some Olig2PC-Astros (6 out of 10) but not in NPC-Astros shown by the traces highlighted in red and enlarged in the insets. The traces are presented after leak subtraction to reveal the voltage-gated currents. ( j ) Current-voltage relationship of the outward currents. ( k ) Using Cs + internal solution, the outward current is eliminated. The inward currents in Olig2PC-Astros are then recorded with the cells held at −70 mV. To maximally activate the inward currents, a 100-ms preconditioning pulse at −100 mV is delivered to the recorded cells before voltage steps (stepped from −70 to +50 mV at 10 mV increments for 50 ms). The representative traces show that the inward currents are reversibly blocked by TTX. The traces are presented after leak subtraction. Student’s t -test, * P <0.05, ** P <0.01 and *** P <0.001. NS represents no significance. Data are presented as mean±s.e.m. Full size image A recent study [2] showed that astroglia with specific regional identity could be derived from hPSCs by the treatment of RA and Pur, which are caudalizing and ventralizing factors, respectively. We thus examined the regional identity of Olig2PC-Astros and NPC-Astros. As shown in Fig. 3b , there were more cells expressing the hindbrain/spinal cord-specific marker HOXB4 in Olig2-Astros than in NPC-Astros ( Fig. 3e , 13±3.2% and 0.9±0.8% for Olig2-Astros and NPC-Astros, respectively; P <0.05, n =4). Notably, the majority of both Olig2-Astros and NPC-Astros expressed the mid/forebrain marker OTX2 ( Fig. 3c and e , 79.2±5.5% and 89.8±4.0% for Olig2-Astros and NPC-Astros, respectively; P >0.05, n =4). A small percent of both Olig2-Astros and NPC-Astros expressed the ventral marker NKX2.1 ( Fig. 3d , 20.2±2.8% and 17±2.7% for Olig2-Astros and NPC-Astros, respectively; P >0.05, n =4). Thus, the majority of both Olig2PC-Astros and NPC-Astros consist of astroglia with the mid/forebrain identity. We also observed that both types of the cells were highly proliferative when cultured in media containing BMP4 or FBS. The proliferation rates of both types of the cells were higher when cultured in the presence of FBS, compared to those of cells when cultured in the presence of BMP4 ( Fig. 3f , P <0.001, n =4). However, NPC-Astros were more proliferative than Olig2PC-Astros when cultured with BMP4 or FBS ( Fig. 3f , P <0.001, n =4). One critical function of astrocytes is to remove glutamate released during neuronal excitation to maintain the normal function of neurons. We thus quantified expression of mRNAs encoding the astrocyte-specific glutamate transporters GLAST and GLT-1 in both astroglial preparations. GLT-1 was expressed at a relatively low level in both astroglia, but GLAST was expressed at much higher abundance in NPC-Astros than in Olig2PC-Astros ( Fig. 3g , P >0.05 for GLT-1 and P <0.01 for GLAST, respectively, n =3 for both genes). Both astroglial populations were competent to take up glutamate from the medium in a sodium- and time-dependent manner ( Fig. 3h ). Consistent with the qPCR data indicating that NPC-Astros expressed higher level of GLAST gene, NPC-Astros showed glutamate uptake at a higher rate at the 30-min time point than Olig2PC-Astros ( Fig. 3h , P <0.05, n =4), but when the incubation time was extended to 60 min, both astroglia reached similar efficiency in glutamate uptake ( Fig. 3h , P >0.05, n =4). Astroglia cells are also heterogeneous in electrophysiological properties. A sustained outward current was recorded from both astroglia ( Fig. 3i ), and this current was eliminated by replacing internal K + with Cs + ( Fig. 3k ), indicating that this current was carried by K + . The current–voltage relationship is shown in Fig. 3j . Interestingly, we observed a small inward current in some Olig2PC-Astros ( Fig. 3i inset, 6 out of 10) upon depolarization, but no inward current was detected in any NPC-Astros. A previous study [32] demonstrated the expression of voltage-gated sodium channel in human astrocytes. To further examine the nature of the inward current, we recorded Olig2PC-Astros using Cs + internal solution, and preconditioned the cells at −110 mV before voltage steps. As shown in Fig. 3k , the inward currents were successively activated upon depolarization and reversibly blocked by TTX, indicating that the currents were mediated by voltage-gated sodium channel. However, no action potentials could be elicited under the current clamp from both astroglia. Thus, both astroglia expressed functional voltage-gated potassium channels, and Olig2PC-Astros differed from NPC-Astros by exhibiting small inward voltage-gated sodium currents. Interaction of the astroglia with neurons in vitro Astrocytes are known to secrete factors that powerfully induce the formation of excitatory synapses between CNS neurons [33] . To examine whether Olig2PC-Astros and NPC-Astros have such effects, we fed primary mouse hippocampal neurons with astroglial cell-conditioned medium (ACM). As shown in Fig. 4a , the miniature excitatory postsynaptic currents (mEPSCs) were recorded from neurons fed with or without concentrated ACM. Interestingly, the addition of ACM from either Olig2-Astros or NPC-Astros significantly increased the amplitude of the mEPSCs ( Fig. 4b and d , n =7, P <0.05), but did not change the frequency of the mEPSCs ( Fig. 4c , n =7, P >0.05). Many factors are known to be secreted by astrocytes and are critical for regulating synapse formation and function, such as apolipoprotein E (APOE), amyloid precursor protein (APP), thromobospondins (TSPs) and glypicans (GPCs) [34] , [35] , [36] . We found that mRNAs encoding TSP-1, APOE, GPC4 and GPC6 were expressed at a much higher level in Olig2PC-Astros than in NPC-Astros ( Fig. 4e , P <0.001 for TSP-1, n =3; P <0.01 for APOE, GPC4 and 6, n =3), whereas mRNA encoding TSP-2 was expressed at higher level in NPC-Astros than in Olig2PC-Astros ( Fig. 4e , P <0.001, n =3). The expression level of APP mRNA was not significantly different between the two astroglia ( Fig. 4e , P >0.05, n =3). 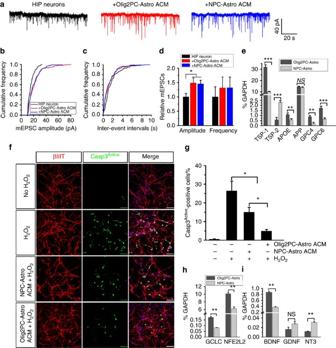Figure 4: Effects of ACM from Olig2PC-Astros and NPC-Astros on neurons. (a) Examples of mEPSC recordings from primary hippocampal (HIP) neurons and HIP neurons fed with ACM from Olig2PC-Astros or NPC-Astros. (bandc) Normalized cumulative curves showing the effects of ACM on the amplitude and frequency of mEPSCs from the sample neurons. (d) Statistical results demonstrating that the amplitude is significantly increased by adding ACM from both Olig2PC-Astros and NPC-Astros, but the frequency is not changed. Each column represents the averaged value from seven neurons (n=7). (e) RT-PCR analysis of the expression of the genes encoding factors that are crucial for regulating synapse formation and function, which includes TSP-1 and 2, APOE, APP and GPC4 and 6. (f) βIII tubulin and activated caspase-3 co-staining of hESC-derived neurons treated with medium alone or medium plus H2O2, NPC-Astro ACM plus H2O2and Olig2PC-Astro ACM plus H2O2. Blue, DAPI-stained nuclei. Scale bars represent 50 μm. (g) Quantification of βIII tubulin+and activated caspase-3+cells among the groups with different treatments (n=4). One-way ANOVA test; *P<0.05. (handi) RT-PCR analysis of the expression of the antioxidant defense-related genes, GCLC and NFE2L2 (n=3), and the neurotrophic growth factor genes, BDNF, GDNF and NT-3 (n=3). Student’st-test; *P<0.05, **P<0.01 and ***P<0.001. NS represents no significance. Data are presented as mean±s.e.m. Figure 4: Effects of ACM from Olig2PC-Astros and NPC-Astros on neurons. ( a ) Examples of mEPSC recordings from primary hippocampal (HIP) neurons and HIP neurons fed with ACM from Olig2PC-Astros or NPC-Astros. ( b and c ) Normalized cumulative curves showing the effects of ACM on the amplitude and frequency of mEPSCs from the sample neurons. ( d ) Statistical results demonstrating that the amplitude is significantly increased by adding ACM from both Olig2PC-Astros and NPC-Astros, but the frequency is not changed. Each column represents the averaged value from seven neurons ( n =7). ( e ) RT-PCR analysis of the expression of the genes encoding factors that are crucial for regulating synapse formation and function, which includes TSP-1 and 2, APOE, APP and GPC4 and 6. ( f ) βIII tubulin and activated caspase-3 co-staining of hESC-derived neurons treated with medium alone or medium plus H 2 O 2 , NPC-Astro ACM plus H 2 O 2 and Olig2PC-Astro ACM plus H 2 O 2 . Blue, DAPI-stained nuclei. Scale bars represent 50 μm. ( g ) Quantification of βIII tubulin + and activated caspase-3 + cells among the groups with different treatments ( n =4). One-way ANOVA test; * P <0.05. ( h and i ) RT-PCR analysis of the expression of the antioxidant defense-related genes, GCLC and NFE2L2 ( n =3), and the neurotrophic growth factor genes, BDNF, GDNF and NT-3 ( n =3). Student’s t -test; * P <0.05, ** P <0.01 and *** P <0.001. NS represents no significance. Data are presented as mean±s.e.m. Full size image A recent study [30] showed that astroglia derived from hESCs promoted the protective effects on hESC-derived neurons against oxidative damage through the release of soluble factors. We thus examined neuroprotective effects of the ACM from both astroglia on hESC-derived neurons, using H 2 O 2 to model an oxidative insult. We quantified the cell death in response to H 2 O 2 treatment by co-staining of activated caspase-3 and βIII-tubulin. As shown in Fig. 4f , treatment of neurons with 50 μM H 2 O 2 caused an increase in active caspase-3-positive neurons from 0.5±0.3% to 26.4±5.2% ( n =4). Addition of ACM from either NPC-Astros or Olig2PC-Astros resulted in significant neuroprotective effects against H 2 O 2 -induced injury, compared to unconditioned medium ( Fig. 4f and g , P <0.05, n =4). Interestingly, Olig2PC-Astro ACM exhibited a neuroprotective effect significantly superior to NPC-Astro ACM ( Fig. 4g , the percentage of active caspase-3 positive neurons were 6.1±1.3% for Olig2PC-Astro ACM and 13.4±2.6% for NPC-Astros ACM, respectively, P <0.05, n =4). Activation of nuclear factor-erythroid 2-related factor 2 (Nrf2) in astrocytes conferred increased antioxidant capacity on neurons during brain ischaemia [37] , [38] . We therefore quantified the expression of two Nrf2 target genes, NFE2L2 (encoding Nrf2 itself) and the glutamate-cysteine ligase catalytic subunit (GCLC), in both astroglia. Compared to NPC-Astros, Olig2PC-Astros showed much higher basal levels of both NFE2L2 and GCLC, indicative of a higher basal Nrf2 activity ( Fig. 4h , P <0.01, n =3 for both genes). We also examined the expression level of the neurotrophic factors BDNF, GDNF and NT-3 in both astroglia. As shown in Fig. 4i , BDNF mRNA was expressed at a much higher level in Olig2PC-Astros than in NPC-Astros. NT-3 mRNA was expressed at low levels in both astroglia, but the expression was higher in NPC-Astros than in Olig2PC-Astros ( Fig. 4i , P <0.01, n =3 for both genes). The expression level of GDNF mRNA was not significantly different between the two astroglia ( Fig. 4i , P >0.05, n =3). Neuroprotection of the grafted astroglia in vivo GCI occurs in patients with a variety of clinical conditions including cardiac arrest and shock, and in patients undergoing complex cardiac surgery. Transient GCI in the rat model leads to delayed and selective neuronal death of pyramidal neurons in the hippocampal CA1 region, which provides us with a time window to perform transplantation study and allows us to examine the neuroprotective effects of transplanted cells on the CA1 neurons. We transplanted the astroglia cells into the left ventricle 6 h after GCI. One or 2 weeks later, no tumour formation or overgrowth of the transplanted cells was observed. As shown in Fig. 5a–c , at 7 days after transplantation, both Olig2PC-Astros and NPC-Astros survived in the rat brain and were identified by human nuclei (hN) and human mitochondria (hM) staining. The majority of the transplanted astroglia were found around the injection site and migrated into the corpus collasum. The transplanted astroglia were also labelled by human CD44 ( Fig. 5d ). They accumulated in the lateral ventricle and some of the cells migrated to the hippocampus ( Fig. 5e and Supplementary Fig. S4a ). In the hippocampal CA1 region, the transplanted astroglia were identified by hN staining ( Fig. 5g and Supplementary Fig. S4b ). As shown in Fig. 5f , the engraftment efficiency was indistinguishable between Olig2PC-Astro and NPC-Astro transplantation groups. On that basis, we further assessed the neuroprotective effects of the transplanted astroglia. At 2 weeks after transplantation, many of the transplanted cells were still found in the CA1 region ( Fig. 6 ). The vast majority of the transplanted cells retained an astroglial phenotype in the ischaemic brain, as indicated by the double-labeling of S100β/hM staining ( Fig. 6a and e , 87.7±3.1% and 89.1±2.8% of hM + cells are S100β + for NPC-Astros and Olig2PC-Astros, respectively; n =7–8). Although positive for GFAP in vitro , the NPC-Astros and Olig2PC-Astros did not strongly express GFAP in vivo after transplantation, as indicated by the double-labeling of GFAP/hN ( Fig. 6b and b , 53.8±4.9% and 63.9±9.2% of hN + cells are GFAP + for NPC-Astros and Olig2-Astros, respectively; n =7–8). At 2 weeks after GCI, we observed the activation of endogenous astrocytes and hypertrophy with increased GFAP staining in CA1 region ( Fig. 6b , upper panels). Interestingly, the transplanted astroglia suppressed GFAP expression, suggesting the suppression of the activation of endogenous astrocytes ( Fig. 6b , middle and lower panels). None of the transplanted astroglia became OPCs or neurons, as indicated by lack of double-labeling for hN and NG2 or hM and NeuN ( Supplementary Fig. S5 ). 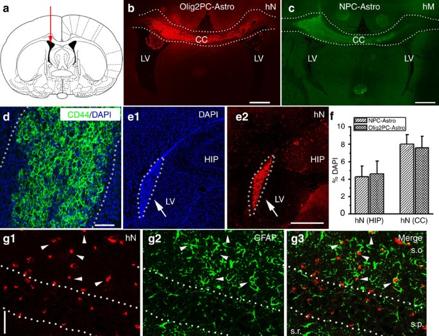Figure 5: Transplantation of human astroglia into rat brains subjected to GCI. (a) Diagram showing the intraventricular transplantation site. (bandc) Representative images showing that at 7 days after transplantation, the transplanted Olig2PC-Astros (b) and NPC-Astros (c) were identified by human nuclei (hN) and human mitochondria (hM) staining. Notably, the majority of the transplanted astroglia were found around at the injection site and the corpus collusum (CC). Dotted lines highlight CC. LV: lateral ventricle. Scale bars represent 100 μm. (d) A representative image from Olig2PC-Astro transplantation group showing that the transplanted astroglia were also labelled by human CD44. Dotted lines highlight CC. Blue, DAPI-stained nuclei. Scale bar represents 50 μm. (e1–2) The transplanted Olig2PC-Astros were also found in the ventricle and the hippocampus (HIP) region. Dotted lines highlight that some of the transplanted Olig2PC-Astros accumulated in the LV. e1, DAPI; e2, hN. Scale bar represents 100 μm. (f) Quantitative results from brain sections containing structures of the HIP and CC showing that no difference in engraftment success (hN+cells) was noted between Olig2PC-Astro and NPC-Astro transplantation groups (n=7–8). Data are represented as mean±s.e.m. (g1–3) Representative images from the hippocampal CA1 region showing that the transplanted Olig2PC-Astros migrate into the CA1 region and express GFAP. d1, hN; d2, GFAP. Arrowheads in d3 indicate the cells double labelled with hN and GFAP. s.o., stratum oriens; s.p., stratum pyramidale and s.r., stratum radiatum. Scale bar represents 50 μm. Figure 5: Transplantation of human astroglia into rat brains subjected to GCI. ( a ) Diagram showing the intraventricular transplantation site. ( b and c ) Representative images showing that at 7 days after transplantation, the transplanted Olig2PC-Astros ( b ) and NPC-Astros ( c ) were identified by human nuclei (hN) and human mitochondria (hM) staining. Notably, the majority of the transplanted astroglia were found around at the injection site and the corpus collusum (CC). Dotted lines highlight CC. LV: lateral ventricle. Scale bars represent 100 μm. ( d ) A representative image from Olig2PC-Astro transplantation group showing that the transplanted astroglia were also labelled by human CD44. Dotted lines highlight CC. Blue, DAPI-stained nuclei. Scale bar represents 50 μm. ( e 1–2) The transplanted Olig2PC-Astros were also found in the ventricle and the hippocampus (HIP) region. Dotted lines highlight that some of the transplanted Olig2PC-Astros accumulated in the LV. e1, DAPI; e2, hN. Scale bar represents 100 μm. ( f ) Quantitative results from brain sections containing structures of the HIP and CC showing that no difference in engraftment success (hN + cells) was noted between Olig2PC-Astro and NPC-Astro transplantation groups ( n =7–8). Data are represented as mean±s.e.m. ( g 1–3) Representative images from the hippocampal CA1 region showing that the transplanted Olig2PC-Astros migrate into the CA1 region and express GFAP. d1, hN; d2, GFAP. Arrowheads in d3 indicate the cells double labelled with hN and GFAP. s.o., stratum oriens; s.p., stratum pyramidale and s.r., stratum radiatum. Scale bar represents 50 μm. 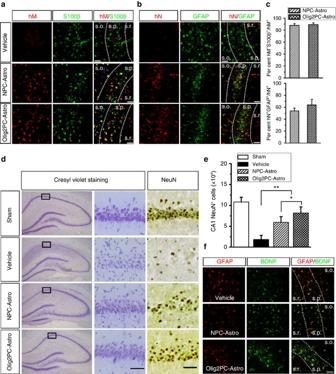Figure 6: Neuroprotective effects of NPC-Astros and Olig2PC-Astros following GCI. (aandb) After being transplanted intraventricularly, both Oilg2PC-Astro and NPC-Astro were identified by anti-hN or anti- hM staining in the hippocampal CA1 region. The majority of Olig2PC-Astros and NPC-Astros were also positive for the astroglial markers S100β (a) and GFAP (b). Notably, the GFAP expression by endogenous gliosis in the GCI injury model was suppressed by the transplant astroglia, compared to the vehicle group (right panels). Scale bars represent 20 μm. (c) Quantification of the percentage hM+S100β+or hN+GFAP+in hM+or hN+transplanted astroglia, respectively (n=7–8). (d) Representatives of cresyl violet staining and NeuN DAB staining performed on the sections from the hippocampus in the sham group and groups subjected to 14 days of reperfusion after 15 min of GCI with vehicle control and intraventricular administration of NPC-Astros or Olig2-Astros 6 h after ischaemia. The squared areas in cresyl violet staining are shown in high magnification. Correspondent areas were also shown for NeuN staining. Scale bars represent 50 μm. (e) The number of hippocampal CA1 neurons in the different groups measured by stereological analysis (n=6 for each group). (f) Representatives of BDNF expression (green) in the hippocampal CA1 region from vehicle group and groups received astroglial transplants. Astrocytes are labelled by GFAP (red) in the different groups. Scale bars represent 20 μm. One-way ANOVA test; **P<0.01, *P<0.05. Data are presented as mean±s.e.m. Full size image Figure 6: Neuroprotective effects of NPC-Astros and Olig2PC-Astros following GCI. ( a and b ) After being transplanted intraventricularly, both Oilg2PC-Astro and NPC-Astro were identified by anti-hN or anti- hM staining in the hippocampal CA1 region. The majority of Olig2PC-Astros and NPC-Astros were also positive for the astroglial markers S100β ( a ) and GFAP ( b ). Notably, the GFAP expression by endogenous gliosis in the GCI injury model was suppressed by the transplant astroglia, compared to the vehicle group (right panels). Scale bars represent 20 μm. ( c ) Quantification of the percentage hM + S100β + or hN + GFAP + in hM + or hN + transplanted astroglia, respectively ( n =7–8). ( d ) Representatives of cresyl violet staining and NeuN DAB staining performed on the sections from the hippocampus in the sham group and groups subjected to 14 days of reperfusion after 15 min of GCI with vehicle control and intraventricular administration of NPC-Astros or Olig2-Astros 6 h after ischaemia. The squared areas in cresyl violet staining are shown in high magnification. Correspondent areas were also shown for NeuN staining. Scale bars represent 50 μm. ( e ) The number of hippocampal CA1 neurons in the different groups measured by stereological analysis ( n =6 for each group). ( f ) Representatives of BDNF expression (green) in the hippocampal CA1 region from vehicle group and groups received astroglial transplants. Astrocytes are labelled by GFAP (red) in the different groups. Scale bars represent 20 μm. One-way ANOVA test; ** P <0.01, * P <0.05. Data are presented as mean±s.e.m. Full size image To ascertain whether transplanted astroglia protected CA1 neurons, we evaluated the histology of cresyl violet staining and NeuN-positive hippocampal CA1 neurons. As shown in Fig. 6d , most of the CA1 pyramidal neurons in vehicle control rats had pyknotic and shrunken nuclei, indicating dramatic neuronal loss in the CA1 region by 2 weeks after GCI. We assessed the number of NeuN + neurons in the hippocampal CA1 region by stereology. Both astroglia significantly protected CA1 neurons ( Fig. 6e , P <0.01, compared to the vehicle group, n =6). Notably, Olig2PC-Astros exhibited significantly better neuroprotective effects than NPC-Astros ( Fig. 6e , 81,530±14,930 and 59,400±13,680 for Olig2PC-Astro and NPC-Astro groups, respectively; P <0.05, n =6). As shown in Fig. 5g , the transplanted astroglia, especially Olig2PC-Astros markedly increased BDNF immunoreactivity in the hippocampal CA1 region, which may contribute to the protective effects on neurons against ischaemic injury [39] , [40] . The majority of the GFAP-positive cells were also positive for BDNF staining ( Fig. 5g ), suggesting that both transplanted astroglia and endogenous astrocytes are sources for the BDNF. Grafted astroglia improve behavioural recovery Reactive synaptogenesis evaluated by staining of presynaptic protein synapsin-1 was seen in the hippocampus after brain ischaemia and was seen as an indication to reconstruct the injured neural circuit [41] . Prompting reactive synaptogenesis tremendously improved functional recovery [42] . Consistently, there was significant reactive synaptogenesis in the CA1 region in the GCI model, indicated by quantification of fluorescence intensity of synapsin-1 staining ( Fig. 7a , P <0.05, n =6). Interestingly, transplantation of Olig2PC-Astro further increased the reactive synaptogenesis ( Fig. 7b , P <0.05, n =6). There was a trend of increase in synapin-1 staining in the group that received NPC-Astro transplants, but it was not significantly different from the vehicle group ( Fig. 7b , P >0.05, n =6–8). Accompanying the CA1 neuronal loss, we also observed severe disruption of myelin integrity in the CA1 region, as indicated by myelin basic protein (MBP) staining ( Fig. 7a ). Quantification of fluorescence intensity of MBP staining revealed that both astroglia significantly preserved myelin integrity, and Olig2PC-Astros showed protective effects superior to NPC-Astros ( Fig. 7c , P <0.05, n =6–8). It is unlikely that Olig2PC-Astros and NPC-Astros differentiated to the oligodendroglial lineage and contributed to myelination after transplantation as none of the transplanted astroglia expressed the oligodendroglial progenitor marker NG2 ( Supplementary Fig. S5 ). 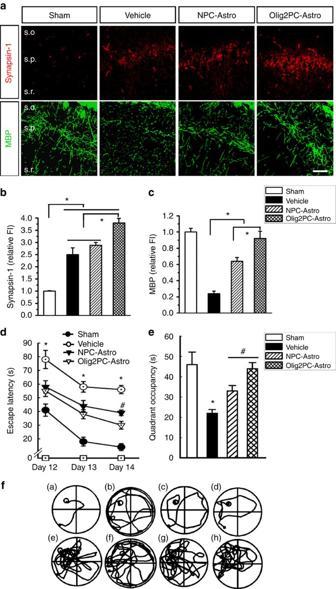Figure 7: The effects of transplanted astroglia on behavioural recovery after GCI. (a) Representatives of synapsin-1 (upper panels) and MBP (lower panels) staining performed on sections from sham, vehicle and groups received Olig2PC-Astro and NPC-Astro transplant. Scale bars represent 20 μm. (bandC) Quantitative analysis of the fluorescence intensity of the synapsin-1 and MBP staining in the CA1 region from the different groups (n=6–8). Note that Olig2PC-Astros has significantly superior effects on promoting reactive synaptogenesis and preserving myelin. One-way ANOVA test; *P<0.05. (d) Morris water-maze task is performed to test the spatial learning ability of the sham, vehicle, and NPC-Astro and Olig2PC-Astro transplanted groups, as shown by the time (escape latency) to find the submerged platform at day 12, 13 and 14 after cerebral ischaemic reperfusion (n=6–8). (e) Probe trials are performed 4 h after the last maze trails on day 14, monitored by relative radial-quadrant occupancy (time spent in the target radial-quadrant). Note that on day 14, animals received NPC-Astros spend significantly more time to find the hidden platform and less time in the target radial-quadrant, compared to the animals received Olig2PC-Astros (n=6–8). (f) Representative sample paths from the maze trials (a–d) and the search patterns on the probe trials (e–h) at 14 days after reperfusion. ((a,e): sham; (b,f): vehicle; (c,g): NPC-Astro transplanted group; (d,h): Olig2PC-Astro transplanted group). Two-way ANOVA test; *P<0.05, comparison between the sham versus and groups received cell transplants; Two-way ANOVA test;#P<0.05, comparison between the two groups received cell transplants. Data are represented as mean±s.e.m. Figure 7: The effects of transplanted astroglia on behavioural recovery after GCI. ( a ) Representatives of synapsin-1 (upper panels) and MBP (lower panels) staining performed on sections from sham, vehicle and groups received Olig2PC-Astro and NPC-Astro transplant. Scale bars represent 20 μm. ( b and C ) Quantitative analysis of the fluorescence intensity of the synapsin-1 and MBP staining in the CA1 region from the different groups ( n =6–8). Note that Olig2PC-Astros has significantly superior effects on promoting reactive synaptogenesis and preserving myelin. One-way ANOVA test; * P <0.05. ( d ) Morris water-maze task is performed to test the spatial learning ability of the sham, vehicle, and NPC-Astro and Olig2PC-Astro transplanted groups, as shown by the time (escape latency) to find the submerged platform at day 12, 13 and 14 after cerebral ischaemic reperfusion ( n =6–8). ( e ) Probe trials are performed 4 h after the last maze trails on day 14, monitored by relative radial-quadrant occupancy (time spent in the target radial-quadrant). Note that on day 14, animals received NPC-Astros spend significantly more time to find the hidden platform and less time in the target radial-quadrant, compared to the animals received Olig2PC-Astros ( n =6–8). ( f ) Representative sample paths from the maze trials (a–d) and the search patterns on the probe trials (e–h) at 14 days after reperfusion. ((a,e): sham; (b,f): vehicle; (c,g): NPC-Astro transplanted group; (d,h): Olig2PC-Astro transplanted group). Two-way ANOVA test; * P <0.05, comparison between the sham versus and groups received cell transplants; Two-way ANOVA test; # P <0.05, comparison between the two groups received cell transplants. Data are represented as mean±s.e.m. Full size image To further explore whether the neuroprotective effects by transplantation of the astroglia could lead to functional improvement, we examined the animals’ learning and memory in Morris water maze. All animals were able to swim normally and locate the hidden platform during the training trials. The time that animals took to locate the platform was measured and shown as escape latency. As expected, rats in the vehicle group had worse performance and required more time to find the platform than those in the sham group. Analysis of escape latency revealed significant differences among vehicle, Olig2PC-Astro and NPC-Astro groups. At the three time points tested, rats in both Olig2PC-Astro and NSC-Astro groups showed less escape latency compared to rats in the vehicle group ( Fig. 7d and f(a–d) , P <0.05, n =6–8). Notably, at day 14, rats in the Olig2PC-Astro group showed better performance compared to rats in the NPC-Astro group ( Fig. 7d , P <0.05, n =6–8). In the probe trials, rats in the sham and both cell transplanted groups showed better performance and spent significantly more time than the vehicle group in the quadrant where the platform had been. Compared to rats in the NPC-Astro group, rats in the Olig2PC-Astro group spent even more time in that quadrant ( Fig. 7e and f(e–h) , P <0.05, n =6–8). Taken together, both grafted astroglia protected the CA1 region after GCI and importantly improved performance in the Morris water-maze test. Notably, Olig2-Astros surpassed NPC-Astros in these protective effects and behavioural improvements. Gene expression analysis of secreted factors To further study the possible mechanisms underlying the superior neuroprotective effect of Olig2PC-Astros, we performed global gene expression microarray. The correlation coefficient ( R 2 ) for genes expressed in NPC-Astros and Olig2-Astros was as high as 0.92 ( Fig. 8a ), indicating the similarity of the two populations. Consistently, Venn diagram ( Fig. 8b ) also revealed that as high as 84.6% of the genes (12,570 out of a total 14,858 transcripts with a detection P -value of ≤0.01) were commonly expressed in both astroglial populations; only 9.3% (1,377 of 14,858) and 6.1% (911 of 14,858) of the genes were uniquely expressed in NPC-Astros and Olig2PC-Astros, respectively. We then focused on analyzing the gene transcripts encoding secreted factors, including neurotrophic factors, BMPs, growth factors, cytokines and chemokines, Wnt ligands, and TNFs. The detailed information of these genes is shown in Supplementary Table S1 . Heat maps in Fig. 8c showed the gene transcripts expressed at higher levels in Olig2PC-Astros than in NPC-Astros, and heat map in Fig. 8d showed the gene transcripts expressed in the opposite situation. Notably, the expression of gene transcripts for BDNF, TSP-1 and 2, NT-3, and GPC4 and 6 were consistent with the qPCR results shown in Fig. 4d and i . Although some gene transcripts related to neuroprotection were expressed at higher levels in NPC-Astros, such as NT-3, TSP-2, Wnt ligands and TNFs, there were more such gene transcripts expressed at higher levels in Olig2PC-Astros, including BDNF, growth factors (FGFs, PDGFs and VEGFs), BMPs and chemokines and cytokines (CLCXs and IL-6). The differential gene expression of secreted factors may collectively account for the compositively superior neuroprotective and behavioural recovery effects of the grafted Olig2PC-Astros, consistent with the previously reported neuroprotective effects of the secreted factors summarized in Supplementary Table S1 . 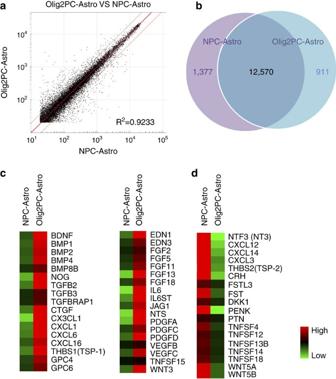Figure 8: Gene expression analysis of NPC-Astros and Olig2PC-Astros. (a) Scatter plot showing the similarity of the NPC-Astro and Olig2PC-Astro populations. (b) Venn diagram showing the number of genes commonly or differentially expressed in the two populations of astroglia. (c–d) Heat maps showing differential gene expression of representative genes encoding factors secreted by NPC-Astros and Olig2PC-Astros. High detection signals relative to the mean were coloured in red. Low detection signals were coloured in green. Figure 8: Gene expression analysis of NPC-Astros and Olig2PC-Astros. ( a ) Scatter plot showing the similarity of the NPC-Astro and Olig2PC-Astro populations. ( b ) Venn diagram showing the number of genes commonly or differentially expressed in the two populations of astroglia. ( c – d ) Heat maps showing differential gene expression of representative genes encoding factors secreted by NPC-Astros and Olig2PC-Astros. High detection signals relative to the mean were coloured in red. Low detection signals were coloured in green. Full size image Here we show that human astroglia generated from hESC-derived Olig2-positive or Olig2-negative neural progenitors are protective against ischaemic brain injury and improve functional outcome. Particularly, by using a comparative approach of engrafting the two different astroglial cell populations, we emphasize the utility of Olig2PC-Astros. Our results further support the notion that not all astroglia cells are equivalent in promoting repair, and suggest that specific populations of astroglia may be of more use than others. Astrocytes are the most numerous cells in the mammalian brain. The complexity and size of human astrocytes are among the few characteristics that differentiate human brains from rodent brains [43] . However, the knowledge on astrocyte development is mainly obtained from rodents. Much remains to be learned about human astroglia development and the heterogeneity of human astrocytes. In this study, using an Olig2-GFP hESC reporter, we demonstrate that human astroglia can be generated from specific neural progenitors, hESC-derived Olig2 + progenitor cells and Olig2 − NPCs. Notably, similar to NPC-Astros, Olig2PC-Astros possess the mid-forebrain or hindbrain/spinal cord identity, suggesting that, like NPCs, Olig2PCs in humans may generate astrocytes throughout the CNS during early development. Previous studies have shown that hESC-derived astroglia can acquire ventral spinal cord identity by the application of morphogens RA and Pur. However, specific concentrations of RA (100 nM) and Pur (~1 μM), and a strict time window of application (over 10-day treatment with RA and Pur starting from neuroepithelial cell stage), are required to fully pattern the neuroepithelial cells and their progeny [2] , [44] . In our differentiation paradigm, treatment of the morphogens RA and Pur did not specify the vast majority of Olig2PC-Astros with a ventral spinal cord identity. We attribute this fact to our specific paradigm of applying the morphogens, in which RA was applied for a short period of time at the embryoid body stage (days 6–10), and Pur was initially applied at a high concentration (1 μM) to induce Olig2 expression (days 6–10) but later applied at a low concentration (0.5 μM) to maintain Olig2 expression in Olig2PCs. Despite the low percentage, there were more Olig2PC-Astros showing spinal cord identity, compared to NPC-Astros. Although possessing many similarities, Olig2PC-Astros are distinct from NPC-Astros in many biological properties including morphology, growth rate, gene expression profile and electrophysiological properties. Together, the differentiation of Olig2PC-Astros and NPC-Astros from hESCs by using different protocols may reflect the fact that human astrocytes are heterogeneous and are derived from distinct progenitors during development. Cell replacement therapy for injured or diseased CNS has promising clinical applications. To date, the types of hPSC derivative cells used for transplantation have ranged from neural stem cells that still have a degree of developmental plasticity, to more restricted neural cells, including various populations of neurons as well as OPCs [45] . However, transplanting hPSC-derived astroglia as a therapeutic strategy has been far less explored. Recent studies [9] , [15] show that transplantation of glial-restricted precursor-derived astroglia promotes functional recovery after spinal cord injury and further suggest that both in vitro astrocytic pre-differentiation and using a specific population of astrocytes (BMP4-induced astrocytes, rather than CNTF-induced astrocytes) are crucial to achieve the regenerative effects. In light of these crucial points, we first differentiated the hESCs to either Olig2-negative NPCs or a pure progenitor population, Olig2PCs, and then induced them to astroglia by BMP4 in high purity under chemically defined and serum-free conditions. Importantly, when intraventricularly transplanted into the brain after GCI, the Olig2PC-Astros and NPC-Astros significantly protected against the CA1 neuronal loss and preserved myelin integrity. The Olig2PC-Astros and NPC-Astros are capable of taking up glutamate and protecting neurons from oxidative stress, which may underlie their protective effects against ischaemic injury as glutamate excitotoxicity and oxygen free radicals are major mechanisms underlying GCI damage [46] , [47] . The transplanted astroglia also increased the reactive synaptogenesis after GCI, as indicated by synapsin-1 staining. A recent study [48] shows that immature rodent astrocytes promote reactive synaptogensis and that astrocyte-secreted TSPs have important roles in this effect. Our in vitro data also demonstrated that both astroglia highly expressed the genes encoding the factors that are crucial for regulating synapse formation and function, including TSPs. Moreover, addition of ACM promoted the synaptic neurotransmission of primary hippocampal neurons. Transplantation of immature astrocytes [5] , [6] has been reported to suppress glia scar formation in the lesioned CNS. The hESC-derived astroglia in this study were at an immature stage and after transplantation, they suppressed the activation of endogenous astrocytes. The Morris water-maze test further demonstrated that the transplanted astroglia also significantly protected spatial learning and memory. Taken together, these results support the potential of using astroglial transplants as cell therapy for ischaemic brain injury. We observed that Olig2PC-Astros showed better neuroprotective effects than NPC-Astros. Moreover, rats that received Olig2PC-Astros exhibited better behavioural recovery after GCI than rats that received NPC-Astros. Mechanistically, we attribute the behavioural improvements to the neuroprotective effects from the transplanted astroglia and the factors released by the two types of astroglia, as implicated by the differential expression of genes encoding growth factors, neurotrophic factors, cytokines and chemokines and factors related to synapse formation and function. The in vivo data further demonstrate that Olig2PC-Astros have superior effects over NPC-Astros in increasing the neurotrophic activity in CA1 region. Olig2PC-Astros may prove to be more useful than NPC-Astros for promoting neurological repair. Our study has thus emphasized the repair potential of astroglia and especially subtype-specific differentiation of astroglia from a pure population of progenitors for optimal outcome in neural repair. In the future, it is important to expand upon our findings to explore the effects of the Olig2PC-Astros derived from human iPSCs. It is also important to examine whether transplantation of Olig2PC-Astros could be beneficial to other CNS injury models, such as focal cerebral ischaemia and CNS traumatic injury models. Ultimately, advancing techniques of isolating characterized unique glial cell types could have tremendous implications for possible therapeutic interventions following CNS damage. Olig2-GFP hESC culture and differentiation Olig2-GFP hESCs were maintained on irradiated mouse embryonic fibroblasts (GlobalStem) in DMEM/F12 medium with 20% knockout serum replacement, 0.1 mM β-mercaptoethanol, 1 × nonessential amino acid, 1 mM L -glutamine (Gibco) and 20 ng ml −1 FGF2 (Millipore) [26] . For feeder depletion, cells were passaged by collagenase (type IV, 1 mg ml −1 ; Invitrogen) treatment, and then hESC colonies were plated on Matrigel (BD Biosciences)-coated plate with mTeSR1 media (STEMCELL Technologies). All experimental procedures conducted on hESCs were approved by the University of California at Davis Stem Cell Research Oversight Committee. To differentiate the Olig2-GFP hESCs to Olig2 + /GFP + progenitor cells, our previous protocol was used with modifications [26] . As shown in Fig. 1a , from days 5 to 9, the EBs were treated with RA (10 μM; Sigma) and Pur (1 μM; Cayman Chemical). At day 9, the EBs were plated onto growth factor-reduced Matrigel (1:30)-coated plates in the presence of Pur (0.5 μM) and the absence of RA. At day 20, the attached EBs became flat and were ready to be disaggregated to single cells using TrypLE (Invitrogen), and were subsequently subjected to FACS based on the GFP fluorescence. To derive NPCs from hESCs, the EBs were plated at day 7 on growth factor-reduced Matrigel-coated plates. NPCs in the form of rosettes were manually picked at day 14 and expanded as neurospheres in a suspension culture in DMEM/F12 medium with 1 × N2 (Invitrogen), 1 × B27-RA (Inivtrogen) and FGF2 (20 ng ml −1 ) until day 20. To further differentiate to astroglia, the FACS-purified Olig2PCs or the NPCs dissociated from the neurospheres at day 20 were attached with a substrate of poly- L -ornithine (0.002%; Sigma) and fibronectin (10 μg ml −1 ; Millipore) in the chemically defined and xeno-free astroglia medium containing DMEM/F12, 1 × N2, 1 × B27-RA, BMP4 (10 ng ml −1 , Peprotech) and FGF2 (20 ng ml −1 ). Both astroglia were maintained in the xeno-free astroglia medium and were only exposed to the medium containing DMEM/F12 and FBS (10%, Invitrogen) to examine the effects of serum on the proliferation and marker expression of both astroglia. For neuronal differentiation, the dissociated NPCs were plated in neuronal differentiation medium containing DMEM/F12, 1 × N2, 1 × B27-RA, 20 ng ml −1 BDNF (Peprotech), 20 ng ml −1 GDNF (Peprotech), 1 mM dibutryrl-cyclic AMP (Sigma) and 200 nM ascorbic acid (Sigma) onto poly- L -ornithine/laminin (50 μg ml −1 )-coated coverslips. The neurons cultured in the neuronal differentiation medium for 4–6 weeks were used for experiments. FACS Sorting of Olig2 + /GFP + cells and data acquisition were performed in a BD FACSCalibur (BD Bioscience). Acquired data were subsequently analyzed by calculating proportions/percentages and average intensities using the FlowJo software (Treestar Inc). Immunostaining Cells fixed with 4% paraformaldehyde and brain sections were processed for immunofluorescence staining [26] . The primary antibodies were listed in Supplementary Table S2 . Coverslips or slides were mounted with the anti-fade Fluoromount-G medium containing 1, 4′,6-diamidino-2-phenylindole dihydrochloride (DAPI) (Southern Biotechnology). Diaminobenzidine (DAB) immunostaining was performed with antibody to NeuN [49] . Images were captured using a Nikon Eclipse C1 confocol laser-scanning microscope or Olympus BX61-DSU microscope. The analysis of fluorescence intensity was performed using ImageJ software. The relative fluorescence intensity was presented as normalized value to the vehicle group. Cell counting and unbiased stereology The cells were counted with ImageJ software (NIH Image). For cultured cells, at least five fields of each coverslip were chosen randomly and three coverslips in each group were counted. For brain sections, an average of three sections was counted per rat spanning 200 μm along the antero-posterior axis. Unbiased stereology was performed on every twentieth section with a distance of 400 μm, located between 2.3 and 4.3 mm posterior to bregma (five to six sections). Cells that are positive for NeuN DAB staining in the hippocampal CA1 region were counted in the serial sections using the optical fractionator counting method [50] in a Stereo Investigator system (MicroBrightField Inc.). The CA1 region was outlined under a × 10 objective of an Olympus microscope. Cell counting was performed with a × 40 objective in fields chosen by the software. The number of cells within the CA1 region on each section was estimated by the Stereo Investigator software [49] . RNA isolation and qPCR RNA was prepared from cell pellets with RNAeasy kit (QIAGEN). Complementary DNA was prepared with a Superscript III First-Strand kit (Invitrogen) [51] . The primers and product sizes are given in Supplementary Table S3 . The PCR products were separated by a 1% agarose gel electrophoresis and visualized by ethidium bromide staining. The qPCR was performed with SYBR GreenER qPCR SuperMix (Life Technologies) or Taqman primers (Life Technologies) on a Roche Lightcycler 480. All experimental samples were analyzed and normalized with the expression level of housekeeping gene Glyceraldehyde-3-phosphate dehydrogenase (GAPDH), n =3 for each. Relative quantification was performed by applying the 2 −ΔΔ C t method [52] . A list of primers is provided in Supplementary Tables S3 and S4 . Images of full-size gels are presented in Supplementary Fig. S6 . Cell proliferation assay Cell proliferation was determined in 96-well plates using MTT (3-(4, 5 dimethylthiazolyl-2)-2,5-diphenyltetrazolium bromide)-based Cell Proliferation Kit I (Roche Diagnostics) [51] . HEK293 cells were used as a normalized control. Glutamate clearance assay The method for measuring the decrease of glutamate over time was modified using the Glutamine/Glutamate Determination Kit (Sigma) [2] . HEK293 cells that do not significantly uptake glutamate compared to primary astrocytes were used as controls. After subtraction of the blanks (0 glutamate added), the decrease in the media, or uptake of glutamate by cells, was reported as μM of glutamate per μg of protein after being normalized to the total protein in each well. The protein content was determined by a BCA protein assay (Pierce). Primary cultur e Primary hippocampal neurons were prepared from C57BL/6 mouse foetuses (Charles River) at embryonic day 15. The hippocampal neurons were cultured with neuron culture medium consisting of Neurobasal medium, 1 × B27(Invitrogen) and cytosine arabionse (1 μM, Sigma) that can eliminate proliferating cells. Starting from DIV 3, the neurons were fed with neuron culture medium alone or neuron culture medium plus concentrated ACM from Olig2PC-Astros or NPC-Astros. The medium was changed every 2 days until experimentation (DIV 8–10). ACM and neuronal injury model ACM was collected using two different methods for different purposes. For preparation of ACM that was used to feed primary hippocampal neurons, both Olig2-Astros and NPC-Astros were cultured in 10-cm plates in astroglia differentiation medium. Then, the cells were plated in minimal condition medium containing phenol-red-free DMEM/F12 and glutamine. After 4 days, ACM was collected, cell debris were pelleted (4 °C, 3400, r.p.m. for 10 min) and then placed in centrifugal concentrators (Millipore) with a size cutoff filter of 3 kDa [36] . ACM was concentrated 50-fold. Protein concentration was determined by Bradford assay, and ACM was fed to primary hippocampal neurons at 100 μg ml −1 . For preparation of ACM that was used to protect hESC-derived neurons from oxidative stress, astroglial cells were treated with salt-glucose-glycine (SGG) minimal medium, consisting of SGG supplemented with 10% MEM (Invitrogen) [30] . After 24 h, ACM was collected, cell debris were pelleted and half-supplemented with fresh minimal medium before the addition of H 2 O 2 . For neuronal injury model, hESC-derived neurons were preconditioned in SGG minimal medium for 12 h, before the addition of control or astrocyte-conditioned minimal medium supplemented with H 2 O 2 (50 μM, Sigma). Electrophysiology Whole-cell voltage-clamp recordings were made from the astroglia cells at room temperature. Pipette electrodes (World Precision Instruments) were fabricated with a Narishige PC-10 vertical puller. Membrane currents were measured with a patch-clamp amplifier (Axon 200B, Axon Instruments), sampled and analyzed with a Digidata 1320A interface and a personal computer with Clampex and Clampfit software (version 9.0.1, Axon Instruments). Pipette electrodes had final tip resistances of 4–6 ΩM. In most experiments, 70–90% series resistance was compensated. The external solution consisted of (in mM) NaCl 150, KCl 5, CaCl 2 2, MgCl 2 1, HEPES 10 and glucose 10 (pH 7.4). The internal solution contained (in mM) NaCl 30, KCl 120, MgCl 2 1, CaCl 2 0.5, HEPES 10, EGTA 5 and MgATP 2 (pH 7.2). A leak subtraction algorithm that was based on the input resistance of individual cells was employed to the I/V relationships in order to more clearly detect voltage-gated K + currents in these cells. For recording Na + currents, KCl in internal solution was replaced with equimolar CsCl. The inward voltage-gated Na + current was identified by its sensitivity to specific voltage-gated sodium channel blocker, tetrodotoxin (TTX, 1 μM; Ascent Scientific). For mEPSCs recording, the internal solution contained (in mM) potassium gluconate 120, KCl 10, EGTA 10 and HEPES 10 (pH 7.2). The mEPSCs was recorded from primary hippocampal neurons at DIV 8–10 in the presence of TTX (1 μM) and bicuculline (20 μM, Tocris). The recorded mEPSCs were analyzed using Mini Analysis programme (Synatosoft). Cell transplantation and histology Transplantation and GCI studies were conducted following protocols approved by the Animal Care and Use Committees at the University of California, Davis and the Medical College of Georgia. All adult (3-month-old) Sprague–Dawley male rats (except the sham control) underwent four-vessel occlusion to generate GCI injury [53] . In order to inject large volume of cell suspension and avoid swelling introduced by the grafted cell suspension, we performed intracerebroventricular injection. Both Olig2PC-Astros and NSC-Astros were suspended at a final concentration of 100,000 cell per μl in PBS, and then 5 μl of cells were administered to the left cerebral ventricles of rats 6 h after GCI. Control rats were infused with PBS as vehicle control. One day before GCI, all animals received daily subcutaneous injection of cyclosporine A (Millipore, 10 mg kg −1 day −1 ) for the duration of the study. One or 2 weeks after transplantation or control injection, the brains were processed for immunohistochemistry. For histological assessment, the dissected brain sections were stained with 0.01% ( w / v ) cresyl violet for 10 min, followed by graded ethanol dehydration. Morris water-maze test Twelve days after ischaemia, the Morris water-maze test was performed [54] . Rats were placed in the water by the hand facing the wall at one random start location out of four, and were allowed to find the submerged platform within 90 s. A trial was terminated if the rats were able to find the platform. If the rat did not find the hidden platform within 90 s, it was guided onto the platform with a stick. The rat was allowed to stay on the platform for 30 s before being removed. The training was repeated from each of the four randomized starting locations, and 4 h was allowed between sessions. The latency time and swimming distance were monitored by an overhead video camera and analyzed by an automated tracking system (San Diego Instruments, CA). One hour after the final training trial, each rat was subjected to a probe trial (90 s) in which no platform was present. The rat was placed in the water at the same random start location, and the time spent in the quadrant that formerly contained the platform was recorded to assess the level of spatial bias. Microarray analysis and heat maps Illumina bead array was performed for gene expression analysis. One hundred nanograms of total RNA were used for amplification and hybridization to Illumina Human HT12_V4 (Illumina). Array was performed by the microarray core facility at UTHSC. Array data were processed using Illumina GenomeStudio software (Illumina). The background was subtracted and arrays were normalized using quantile. Gene expression levels were considered significant only when their detection P -value ⩽ 0.01. Detection P -value is calculated by the equation: detection P -value=1−( R / N ), where R is the rank of the z -score of the analytical probes and N is the number of the negative controls. The z -score is often used in the z -test in standardized testing, which is an analogue of the Student’s t -test for a population whose parameters are known. Scatter plot was generated using GenomeStudio. Heat maps of selected signaling pathway related genes were generated using TMEV programme in the TM4 software package. Data analysis All data represent mean±s.e.m. The escape latency in the behavioural training tests was determined by two-way analysis of variance (ANOVA). All other assessments were analyzed using Student’s t- test when only two groups were compared or one-way ANOVA when three or more groups were compared. Accession codes: Microarray data have been deposited in Gene Expression Omnibus under the accession code GSE47515 . How to cite this article: Jiang, P. et al . hESC-derived Olig2 + progenitors generate a subtype of astroglia with protective effects against ischaemic brain injury. Nat. Commun. 4:2196 doi: 10.1038/ncomms3196 (2013).